Hotspot-mediated ultrafast nonlinear control of multifrequency plasmonic nanoantennas Plasmonic devices have a unique ability to concentrate and convert optical energy into a small volume. There is a tremendous interest in achieving active control of plasmon resonances, which would enable switchable hotspots for applications such as surface-enhanced spectroscopy and single molecule emission. The small footprint and strong-field confinement of plasmonic nanoantennas also holds great potential for achieving transistor-type devices for nanoscale-integrated circuits. To achieve such a functionality, new methods for nonlinear modulation are required, which are able to precisely tune the nonlinear interactions between resonant antenna elements. Here we demonstrate that resonant pumping of a nonlinear medium in a plasmonic hotspot produces an efficient transfer of optical Kerr nonlinearity between different elements of a multifrequency antenna. By spatially and spectrally separating excitation and readout, isolation of the hotspot-mediated ultrafast Kerr nonlinearity from slower, thermal effects is achieved. Concentration of electromagnetic radiation into nanometre-sized volumes is one of the major promises of plasmonics [1] , [2] . Subwavelength focusing of energy is of enormous interest for many applications, including coupling of light to single molecules [3] , [4] , field-enhanced spectroscopy and sensing [5] , [6] , [7] , [8] , [9] , photochemistry [10] , nonlinear frequency conversion [11] , [12] and all-optical switching [13] , [14] , [15] , [16] . In analogy with radiowave antennas, plasmonic nanoantennas are designed to optimize the coupling between far-field light and near-field ‘hotspots’ [5] , [17] . Conversively, the coupling between a small particle and a large nanoantenna can be used to increase the dielectric influence of the small sensing element strategically placed in such a hotspot [6] , [7] . The active control of plasmonic resonances using electrical, optical, or mechanical means is an emerging field with huge potential to achieve low-power reconfigurable and ultracompact switching devices. To successfully achieve effective optical control at the single nanoantenna level, new types of nanoscale hybrid nonlinearities have to be devised [11] , [14] , [15] , [16] . One of the largest optical nonlinearities in nanoplasmonics is generated by the metal itself, through a combination of interband excitations [13] , [20] , hot-plasma effects [16] , [21] , [22] , [23] and electronic charging [24] . Although these nonlinearities of the plasmonic metal can be employed for modulation devices, they are generally associated with a considerable thermal loading of the device and are accompanied by slow thermal relaxation effects. Several schemes have been proposed theoretically for active nanoantenna devices coupled to an external Kerr medium [25] , [26] , [27] . Experimentally, such an ultrafast antenna-enhanced Kerr nonlinearity has not yet been reported. Separation of Kerr nonlinearity from the intrinsic plasmonic heating effects is complicated experimentally even when using the above theoretical schemes, as these all rely on resonant pumping of a single plasmonic mode. Therefore, optical excitation always results in a combination of external nonlinearity of the surrounding medium and intrinsic metallic effects [28] , [29] . The origin of different nonlinear contributions in hybrid nanostructures can, in some cases, be identified through their characteristic spectral and temporal signatures [6] , [30] . Here we demonstrate a new route towards resonant nanoplasmonic switching devices by exploiting a plasmonic hotspot to transfer optical nonlinearity in a multifrequency crossed antenna array. Similar multifrequency antennas have been used before as dual-band antennas for spectroscopy [8] , [31] , [32] and have been proven to be very versatile. Our modulation scheme is distinct, as it relies on pumping of the nonlinear medium around a nanoantenna through another spatially and spectrally separate antenna mode. We show that we can individually address and tune the nonlinearities of the Au and of the external medium through differences in their characteristic spectral shape, time dynamics and dependence on antenna parameters. The hotspot provides an efficient transfer of the ultrafast Kerr nonlinearity while simultaneously isolating the nonlinear thermal response of the metal. A spatially and spectrally separate nonlinear excitation and readout is not only of importance for ultrafast switching devices, it may also be crucial, for example, for coupling actively controlled plasmonic hotspots with other temperature-sensitive solid-state systems, such as quantum emitters. In a series of experiments of increasing complexity, we first investigate resonant pumping of the nonlinear indium-tin oxide (ITO) medium using plasmonic dimer nanoantennas. Subsequently, we use crossed multifrequency antenna arrays to demonstrate hotspot-mediated transfer of nonlinearity in the array. The results are compared with numerical model calculations, allowing to separate nonlinear contributions from the metallic system and hotspot-mediated ITO Kerr nonlinearity. Resonant nonlinear control of plasmonic dimer antennas We exploit the unique properties of highly doped metal oxides to mediate the nonlinear interaction between the individual nanoantenna arrays. Highly doped transparent conducting oxides are Drude metals with a free electron density as high as 10 21 cm −3 and an optical response governed by the collective oscillations of the free electron gas. The nonlinear optical response of metal oxides has only recently attracted attention in the context of nanoplasmonics research [12] , [15] , [28] , [29] , [30] , [33] , [34] , [35] . Similar to metals, metal oxides have a large third-order nonlinearity, which can be further sensitized through hybrid interactions with the metal. In our experiments, we investigate gold nanoantennas on a commercial ITO substrate, an arrangement previously used for nonresonant, picosecond pumping [33] . Arrays of plasmonic nanoantennas were fabricated on top of a 120-nm layer of ITO as described in the Methods section. The dimers consist of two closely spaced gold nanorods of varying lengths L ranging from 250 to 450 nm (labelled A–E in Fig. 1 ). A scanning electron microscopy image of the L =250 nm antenna is shown in the inset of Fig. 1a . The main panel of Fig. 1a shows the optical density (OD) of the antenna arrays. All spectra were referenced against the ITO-coated substrate; the extinction of the ITO-coated substrate is given by the black solid line in Fig. 1a . The dipolar antenna mode shifts from 1,050 nm for the L =250 nm antennas to 1,200 nm for the L =450 nm antennas. This trend is reproduced well by numerical simulations of the antenna array, including the substrate as shown in Fig. 1b . Differences in amplitude between calculations and experiments are attributed to inhomogeneous broadening of the experimental data originating from variations in individual shapes and from polycrystallinity of the Au antennas. The resonant response of the dimer antennas results in a local field enhancement in the antenna gap, as is illustrated by the near-field map of Fig. 1b , showing the calculated field for the L =250 nm antenna at a wavelength of 1,030 nm. To assess the resonant response of the different antenna arrays at the fixed pump wavelength, we calculated the plasmonic near-field enhancement at 1,030 nm for both polarizations. 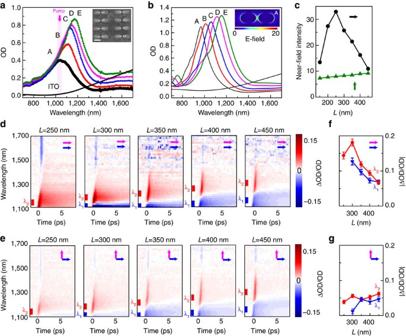Figure 1: Resonant pumping of dimer antennas. Measured (a) and simulated (b) optical density (OD) spectra of arrays A-E of dimer antennas with lengths from 250 nm (A) to 450 nm (E) for polarization along the antenna. Inseta: scanning electron microscopy image of array A; scale bar, 200 nm. Insetb: calculated map of near-field enhancement for antenna A and at the pump wavelength of 1,030 nm. (c) Calculated near-field intensity at 1,030 nm wavelength, at points indicated by white circles in corresponding maps for horizontal polarization (midgap, black dots) and vertical polarization (10 nm above centre of nanorod, green triangles). Pump-probe spectral maps showing nonlinear modulation ΔOD/OD for antenna arrays A-D, for horizontal (d) and vertical (e) pump polarizations. Arrows in each image indicate polarizations of pump (magenta) and probe (blue) with respect to horizontal antenna orientation. (f,g) Maximum |ΔOD/OD| values for the two pump polarizations, error bars indicate experimental error due to instrumental noise. Figure 1c shows the resulting near-field intensities corresponding to the centre of the gap for horizontal polarization and 10 nm away from the top edge of the nanorods for vertical polarization. Compared with the transverse mode, which only weakly depends on antenna length, the longitudinal mode shows a resonant enhancement of the hotspot intensity in the centre of the gap for antenna lengths around 250 nm. Up to ten times higher intensities were found in the gap close to the interface between the gap media and the antenna (see Supplementary Fig. 1 ). Figure 1: Resonant pumping of dimer antennas. Measured ( a ) and simulated ( b ) optical density (OD) spectra of arrays A-E of dimer antennas with lengths from 250 nm (A) to 450 nm (E) for polarization along the antenna. Inset a : scanning electron microscopy image of array A; scale bar, 200 nm. Inset b : calculated map of near-field enhancement for antenna A and at the pump wavelength of 1,030 nm. ( c ) Calculated near-field intensity at 1,030 nm wavelength, at points indicated by white circles in corresponding maps for horizontal polarization (midgap, black dots) and vertical polarization (10 nm above centre of nanorod, green triangles). Pump-probe spectral maps showing nonlinear modulation ΔOD/OD for antenna arrays A-D, for horizontal ( d ) and vertical ( e ) pump polarizations. Arrows in each image indicate polarizations of pump (magenta) and probe (blue) with respect to horizontal antenna orientation. ( f , g ) Maximum |ΔOD/OD| values for the two pump polarizations, error bars indicate experimental error due to instrumental noise. Full size image We measured the ultrafast nonlinear response of the dimer antenna arrays in the wavelength range of 1,100–1,700 nm. For all experiments, the excitation was fixed at a wavelength of 1,030 nm and a fluence of 4 mJ cm −2 . Figure 1d,e shows the time-resolved spectral response for two different pump polarizations parallel (d) and perpendicular (e) to the antenna long axis, while the probe polarization was kept parallel to the antenna. The maps present the measured relative change ΔOD/OD, where we used the total OD, including the ITO substrate. An extensive analysis of the time dynamics using double-exponential decay fits is presented in Supplementary Figs 2 and 3 (see also Supplementary Note 1 ). An initial, fast component with 0.2 ps is followed by a slower tail with a decay time of several picoseconds. As a simple indicator of the total nonlinear response, we show in Fig. 1f,g the maximum |ΔOD/OD| amplitude around zero delay time at the wavelengths of maximum negative and positive modulation λ 1 and λ 2 . For pump polarization along the nanoantenna, we find an enhancement of the nonlinear response for an antenna length around 300 nm, while the perpendicular polarization does not show a strong dependence on antenna length. This resonant enhancement corresponds well with the overlap of the antenna resonance with the pump wavelength in Fig. 1a as well as with the behaviour of the near-field intensity in Fig. 1c . Therefore, we attribute the increase of the ΔOD/OD amplitude to an enhanced nonlinear response by resonant pumping of the longitudinal antenna mode. The full-time dynamics ( Supplementary Figs 2 and 3 ) reveal different contributions at the two wavelengths λ 1 and λ 2 for the ultrafast ( A 1 ) and slow, picosecond ( A 2 ) effects, which indicates the presence of several different contributions to the nonlinear response with characteristic spectral and temporal signatures. The time dynamics of hot-carrier effects in Au can be described by the two-temperature model, which predicts a picosecond electron–phonon thermalization followed by a slow cooling of the system on a time scale of hundreds of picoseconds ( A 0 in our analysis) [21] . We observed an increase of the picosecond decay time τ 2 with increasing signal strength |ΔOD/OD| (see Supplementary Fig. 4 ), which can be attributed to a dependence of the electronic heat capacity of Au on the temperature of the antenna [36] . The increase in electron damping rate confirms that direct, resonant pumping of the antenna results in a significant heat deposition in the metal. Hotspot-mediated nonlinearity of multifrequency antennas Although the experiment on dimer antennas clearly demonstrates the resonant pumping mechanism, analysis of the different nonlinear contributions is limited, as pump and probe resonance conditions cannot be individually tuned. Therefore, the plasmon mode shifts out of the accessible spectral range for the probe for short antenna lengths near resonant pumping. To gain independent control of resonance conditions for excitation and readout, we designed arrays consisting of two different sublattices of perpendicularly oriented gold nanorods of different lengths. In a series of arrays labelled P-T, the length of the horizontal rods (‘antenna 1’) was kept fixed at L =385 nm, while the length of the vertical rods (‘antenna 2’) was varied between 200 and 410 nm, see Fig. 2a . The extinction spectra of the arrays are shown in Fig. 2b,c for, respectively, vertical (b) and horizontal (c) polarizations. The spectra show the longitudinal and transverse modes L 1 , T 1 of the horizontal nanorods and L 2 , T 2 of the vertical nanorods. Good agreement is obtained with numerical calculations as shown in Fig. 2d,e . The antenna dipole resonance L 1 of antenna 1 is fixed at around 1,180 nm wavelength (a small variation arising from coupling effects in the arrays), while the mode L 2 of antenna 2 is tuned from 970 to 1,220 nm. 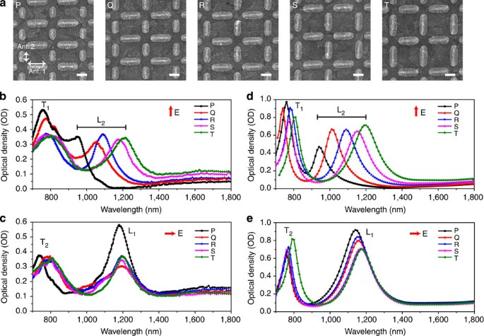Figure 2: Scanning electron microscopy and optical characterization. (a) Scanning electron microscopy images of crossed-antenna arrays P-T used in experiments. Measured (b,c) and simulated (d,e) spectra for light of vertical and horizontal polarization (as indicated by red arrows) for five different arrays of crossed nanoantennas. The size of the horizontal antennas is kept constant at 385 nm, whereas the length of the vertical antennas varies from 200 nm (P) over 260 nm (Q), 300 nm (R), 355 nm (S) and 410 nm (T), which accounts for the observed resonance shift. Figure 2: Scanning electron microscopy and optical characterization. ( a ) Scanning electron microscopy images of crossed-antenna arrays P-T used in experiments. Measured ( b , c ) and simulated ( d , e ) spectra for light of vertical and horizontal polarization (as indicated by red arrows) for five different arrays of crossed nanoantennas. The size of the horizontal antennas is kept constant at 385 nm, whereas the length of the vertical antennas varies from 200 nm (P) over 260 nm (Q), 300 nm (R), 355 nm (S) and 410 nm (T), which accounts for the observed resonance shift. Full size image The crossed antenna design allows selective coupling of light into the two subarrays by controlling the incident polarization. We use this property to investigate the combination of resonant pumping and transfer of nonlinearity by exciting mode L 2 of antenna 2 while monitoring the changes in mode L 1 of antenna 1. 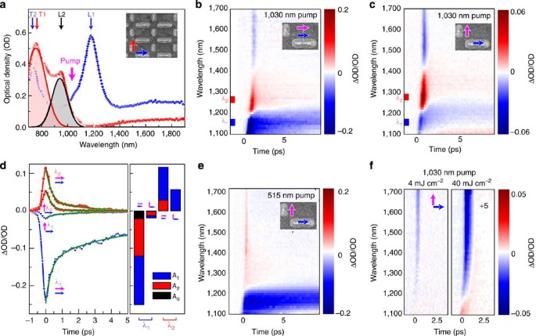Figure 3: Polarization dependence of crossed antenna array. (a) Spectra for crossed antenna array (P) for light polarized in horizontal (blue) and vertical (red) direction. Shaded areas correspond to Gaussian fits of vertically polarized spectra toL2andT1contributions (seeSupplementary Fig. 6). (b,c) Time-dependent pump–probe maps for array P using 1,030 nm wavelength pump and, respectively, horizontal (b) and vertical (c) pump polarization. Probe polarization was kept horizontal. (d) Nonlinear time response (sections of mapsbandc) at selected wavelengthsλ1andλ2, with double exponential decay fits (green lines). Inset shows contributions from ultrafast response (0.2 ps,A1), picosecond dynamics (2–3 ps,A2) and slow cooling (>10 ps,A0) for both pump polarizations. (e) Time-dependent pump–probe maps for array P using 515 nm wavelength pump. (f) Nonlinear response of bare ITO substrate at pump fluences of 4 and 40 mJ cm−2and 1,030 nm wavelength. Figure 3 shows results taken on array P ( L =200 nm). The linear optical spectra for this array in Fig. 3a illustrate several aspects of the experiment. For horizontal pump polarization, antenna 1 is pumped left of the resonance L 1 , which was shown in Fig. 1f to result in off-resonance excitation. For vertical pump polarization, antenna 2 is pumped close to resonance L 2 , which according to Fig. 1f should give a resonant excitation enhancement. For the same polarization, the transverse mode T 1 is pumped far away from its resonance, which is expected to result in an off-resonance component similar to Fig. 1g . Figure 3: Polarization dependence of crossed antenna array. ( a ) Spectra for crossed antenna array (P) for light polarized in horizontal (blue) and vertical (red) direction. Shaded areas correspond to Gaussian fits of vertically polarized spectra to L 2 and T 1 contributions (see Supplementary Fig. 6 ). ( b , c ) Time-dependent pump–probe maps for array P using 1,030 nm wavelength pump and, respectively, horizontal ( b ) and vertical ( c ) pump polarization. Probe polarization was kept horizontal. ( d ) Nonlinear time response (sections of maps b and c ) at selected wavelengths λ 1 and λ 2 , with double exponential decay fits (green lines). Inset shows contributions from ultrafast response (0.2 ps, A 1 ), picosecond dynamics (2–3 ps, A 2 ) and slow cooling (>10 ps, A 0 ) for both pump polarizations. ( e ) Time-dependent pump–probe maps for array P using 515 nm wavelength pump. ( f ) Nonlinear response of bare ITO substrate at pump fluences of 4 and 40 mJ cm −2 and 1,030 nm wavelength. Full size image Figure 3b,c show spectral maps of the time-dependent nonlinear response ΔOD/OD of array P for horizontal (b) and vertical (c) pump polarizations. The time dynamics at selected wavelengths λ 1 and λ 2 , corresponding to the minimum and maximum of nonlinear modulation, respectively, is shown in Fig. 3d . For horizontal pump polarization, a large ΔOD/OD signal is found at λ 1 , comparable to that of the resonant dimer antennas of Fig. 1d . The dynamics were fitted using a double exponential decay yielding amplitudes as indicated in the inset of Fig. 3d . For horizontal pump polarization, the dynamics at λ 1 is characterized by a relatively large contribution of slow, picosecond relaxation processes ( A 2 ) with a long relaxation time τ 2 =3.5±0.2 ps indicative of significant heating. For vertical pump polarization, this λ 1 contribution is strongly suppressed by an order of magnitude and has a relation time τ 2 =2.0±0.1 ps. Compared with this large suppression of nonlinear response at λ 1 , the modulation at λ 2 is only reduced by a factor of 2, mainly due to the suppression of the slow, picosecond component ( A 2 ) in the perpendicular pumping configuration. Next to resonant pumping at 1,030 nm, we investigated nonresonant pumping at a wavelength of 515 nm ( Fig. 3e ). In this case, the gold is heated directly through interband excitations and the response does not depend on pump polarization. Clearly, off-resonance pumping at 515 nm only produces the slow, picosecond component at λ 1 , whereas the contribution at λ 2 is completely absent. We therefore attribute the slow component at λ 1 for all antennas to direct excitation of the Au nanorods. In contrast, the ultrafast component observed at λ 2 in the antenna modulation of both Fig. 3b,c bears close resemblance to the nonlinear modulation observed for the ITO substrate itself in the absence of any antennas ( Fig. 3f ). The pure ITO modulation is also observed for the antenna arrays at wavelengths above 1,400 nm, that is, outside the plasmon resonance band. The ITO substrate could be pumped at significantly higher, nondestructive pump intensities corresponding to 40 mJ cm −2 , resulting in data showing that the nonlinear ITO response actually changes sign at shorter wavelengths ( Fig. 3f ). Further discussion on the nature of the ITO nonlinearity is presented in the modelling section. The comparison of the nonlinear response of crossed arrays with different resonance wavelengths allows a clear separation of the resonant contribution from the hotspot-mediated ITO nonlinearity in the plasmonic modulation, as is shown in Fig. 4a . The analysis of fast and slow dynamics for the crossed antenna arrays is presented in the Supplementary Fig. 5 . 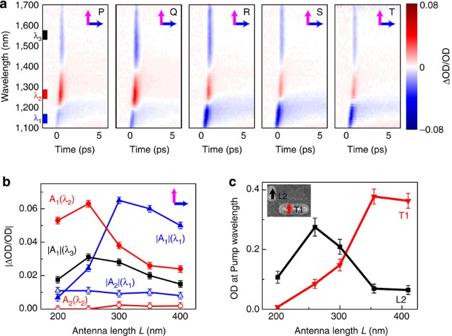Figure 4: Dependence on antenna parameters. (a) Pump–probe measurements for crossed antenna arrays P-T, with scanning electron microscopy images illustrating polarizations of pump and probe. (b) Modulation amplitudes |ΔOD/OD| at selected wavelengthsλ1–λ3, for ultrafast (A1) and picosecond (A2) components. Error bars inbindicate 95% confidence interval of the fits. (c) Values for the OD at the pump wavelength of 1,030 nm extracted by fitting linear spectra with Gaussians (seeSupplementary Fig. 6). Error bars incindicate experimental measurement accuracy combined with error in Gaussian fits. Figure 4b shows the extracted |ΔOD/OD| response at strategic wavelengths λ 1 and λ 2 for the ultrafast component A 1 and the slow, picosecond component A 2 , as well as the amplitude of the ultrafast ITO nonlinearity around λ 3 =1,580 nm. When plotting the data against the length L of antenna 2, we can distinguish two different trends. Wavelengths λ 2 and λ 3 both show a maximum in nonlinear response for array Q ( L =260 nm), while the response at λ 1 shows a completely different trend increasing towards longer antenna lengths. The origin of these two trends can be identified by a more detailed analysis of the absorption spectra for vertical polarization. As indicated in Fig. 3a , we can fit the different modes to Gaussian resonance profiles with good accuracy (results for all arrays are shown in Supplementary Fig. 6 ). This allows us to extract the OD at the pump wavelength of 1,030 nm for both the longitudinal mode L 2 and the transverse mode T 1 . The results of this analysis are plotted in Fig. 4c . Clearly, the modulation at λ 2 and λ 3 follows the absorption of the longitudinal mode of the vertical antenna 2 (the vertical antenna), while the ΔOD/OD at λ 1 can be described well by absorption through the transverse mode of the readout antenna 1 itself. Thus, from Figs 3 and 4 , the following picture emerges: excitation of the readout antenna itself results in a slow, picosecond contribution due to heating of the antenna–ITO hybrid through metal-induced absorption. In addition, a resonant component is found in the response of antenna 1 mediated through cross-excitation of the ITO substrate through the longitudinal mode of the perpendicular antenna 2. Figure 4: Dependence on antenna parameters. ( a ) Pump–probe measurements for crossed antenna arrays P-T, with scanning electron microscopy images illustrating polarizations of pump and probe. ( b ) Modulation amplitudes |ΔOD/OD| at selected wavelengths λ 1 – λ 3 , for ultrafast ( A 1 ) and picosecond ( A 2 ) components. Error bars in b indicate 95% confidence interval of the fits. ( c ) Values for the OD at the pump wavelength of 1,030 nm extracted by fitting linear spectra with Gaussians (see Supplementary Fig. 6 ). Error bars in c indicate experimental measurement accuracy combined with error in Gaussian fits. Full size image Numerical model of nonlinear modulation Our experimental findings are supported by numerical model calculations of the nonlinear response, as is shown in Fig. 5a–d . 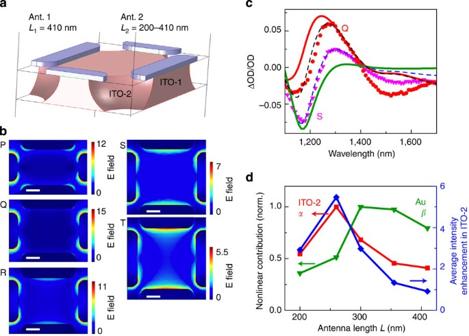Figure 5: Numerical model. (a) Illustration of geometry used in numerical simulations of antenna modulation. ITO-1 and ITO-2 represent different areas of the ITO substrate corresponding to unmodulated substrate and modulated hotspot, respectively. (b) Calculated near-field maps at pump wavelength of 1,030 nm and for vertically polarized excitation, showing resonant enhancement for (vertical) antenna 1 and transverse mode of (horizontal) antenna 2. (c) Fits to ultrafast nonlinear response for arrays Q and S (dashed lines), with symbols showing experimental data. Full lines show maximum individual contributions for electronic heating of Au (green, 20% increase of Drude damping rate of Au antennas) and hotspot-mediated ITO-2 nonlinearity (red, −5% electron density modulation in ITO-2). (d) Normalized nonlinear contributions for the Au (green triangles) and ITO-2 (red squares) components versus lengthL2of antenna 2. Blue diamonds show calculated near-field intensity enhancement averaged over ITO-2 volume. Figure 5a shows a unit cell of the model array, which was positioned on an ITO substrate. Figure 5b shows near-field maps at the pump wavelength of 1,030 nm. A maximum local field enhancement of 15 is found for array Q . To incorporate a local nonlinearity mediated by the longitudinal antenna resonance in a first-order approximation, the substrate was divided into two different regions, corresponding to the bulk of the substrate (ITO-1) and spherical pockets around the endcaps of the antennas (ITO-2, see Fig. 5a ). Subsequently, nonlinear excitation through resonant pumping of antenna 2 was modelled by changing the dielectric function of ITO-2. The nonlinear Kerr effect was modelled as a change in the refractive index of ITO, Δ n , proportional to the product of the third-order susceptibility and the square of the local electric field χ (3) E 2 . In a first approximation, we model the change in ITO response by a constant Δ n within the ITO-2 pockets, which corresponds to assuming a volume averaged homogeneous E 2 in this region. The second source of nonlinearity in the arrays is produced by heating of the gold antennas. This is taken into account by increasing the Drude damping rate in the antenna, which has been shown to be the dominant nonlinearity for Au in the near infrared [21] , [22] . Figure 5: Numerical model. ( a ) Illustration of geometry used in numerical simulations of antenna modulation. ITO-1 and ITO-2 represent different areas of the ITO substrate corresponding to unmodulated substrate and modulated hotspot, respectively. ( b ) Calculated near-field maps at pump wavelength of 1,030 nm and for vertically polarized excitation, showing resonant enhancement for (vertical) antenna 1 and transverse mode of (horizontal) antenna 2. ( c ) Fits to ultrafast nonlinear response for arrays Q and S (dashed lines), with symbols showing experimental data. Full lines show maximum individual contributions for electronic heating of Au (green, 20% increase of Drude damping rate of Au antennas) and hotspot-mediated ITO-2 nonlinearity (red, −5% electron density modulation in ITO-2). ( d ) Normalized nonlinear contributions for the Au (green triangles) and ITO-2 (red squares) components versus length L 2 of antenna 2. Blue diamonds show calculated near-field intensity enhancement averaged over ITO-2 volume. Full size image Previous studies of the Kerr nonlinearity in ITO [37] have identified a relation with a polarization due to free carriers, resulting in a positive real χ (3) . Compared with those earlier studies, our current work involves much higher carrier densities and concomitantly stronger contribution from plasmonic effects. Exactly the same sample conditions were discussed previously related to a much slower, thermo-optic nonlinearity of ITO [33] , where we found a spectral response closely resembling the shape and sign change found in Fig. 3f . Other studies have identified carrier density modulation as the governing nonlinearity of ITO under ultraviolet laser excitation [34] . On the basis of these arguments, we modelled the ITO nonlinear response Δ n through a modulation of the plasmon frequency. We note that this model produces a positive and real Kerr coefficient at frequencies above the bulk plasmon frequency, consistent with results from earlier studies [37] . The individual effects of the two types of nonlinearity are shown in Fig. 5c . The red curve corresponds to the ΔOD/OD response for a 5% reduction of the ITO-2 carrier density. The green curve corresponds to a 20% increase of the Drude damping rate of the Au antennas. These values represent the largest modulations found in our measurements, respectively, for arrays Q and S. Clearly, the ITO-2 nonlinearity contributes mostly to the positive peak at 1,280 nm, while the Au nonlinearity results in the negative plasmon bleaching contribution at 1,180 nm. The combined response of all arrays under study could be fitted to good agreement using a superposition of these two independent contributions using only two scaling parameters α and β according to ΔOD/OD= α ΔOD/OD ITO2 + β ΔOD/OD Au , where correspond to the maximum individual effects as indicated by the red and green curves in Fig. 5c . Figure 5c shows the resulting curves for the two extreme cases corresponding to arrays Q and S, which are respectively given by α Q =1.00, β Q =0.45 and α S =0.45, β S =1.0, respectively. Fits for all other arrays are show in Supplementary Fig. 7 . Above 1,400 nm wavelength, poor agreement is obtained because of the absence of the ITO-1 substrate modulation in our simplified model. The resulting values for α and β for all arrays are shown in Fig. 5d . The ITO-2 contribution to the nonlinear response of antenna 2 correlates well with the volume-averaged near-field enhancement, as shown by the blue diamonds in Fig. 5d . Here we averaged the near-field intensity maps of Fig. 5b over the entire volume of the spherical pocket to obtain an average enhancement factor. Enhancements of up to five times the incident intensity are obtained, which predicts a corresponding enhancement of the nonlinear Kerr effect in the hotspot. Our results on the crossed antenna arrays show a nonlinear contribution on the horizontal antenna 1 mediated by resonant pumping of the vertical antenna 2. Both the nonlinear response of the longitudinal L 1 plasmon mode and of the ITO background show the same resonant dependence on the length of antenna 2, indicating that the ITO substrate mediates the resonant nonlinearity of antenna 1. The numerical simulations provide further evidence that this nonlinearity is induced by the local field enhancement associated with the longitudinal L 2 plasmon mode for the vertical pump, horizontal probe geometry. Although the positive ultrafast modulation at λ 2 is nearly as strong as for the horizontal pump, horizontal probe configuration, the readout antenna suffers less from nonresonant thermal effects. Thus, the cross-excitation scheme allows for a physical separation of the position where excess energy is deposited into the system from the position where modulation takes place. This configuration will be beneficial for applications benefiting from fast, nonthermal nanophotonic switching, where spurious heating effects have to be suppressed. Such nonthermal modulation schemes are of great interest, for example, for the control of nanoscale emitters or other quantum systems. In plasmonic devices, heat deposition through ohmic losses is an inherent property of the scheme. Although these effects cannot be avoided on the systems scale, we show here a new route to locally limit the impact of thermal effects. Our results furthermore demonstrate the potential of highly doped metal oxides as nonlinear materials for ultrafast plasmonic devices. The strong dependence of the nonlinear optical response of the ITO on excitation conditions, and in particular on the pump wavelength, found in this work and elsewhere [33] , [34] invites further studies to identify the underlying mechanisms and dynamics of these highly complex optical materials. Although current work showed significant contributions from excitation through the transverse ( T 1 ) plasmon resonance of the readout antenna, further reduction of thermal effects may be achieved by tuning these modes further away from the excitation wavelength. To enhance the modulation effects, optimization of the nonlinear cross-coupling will be desirable to obtain stronger hotspot intensities and thus a larger transfer of nonlinearity. Here, a balance will have to be found between hotspot-induced Kerr nonlinearities induced by the external gap loading material and the linear interactions between the metal antennas taking place through mode hybridization for small antenna gaps. In particular, the latter will result in polarization conversion and an effective transfer of energy between the two antennas [38] , and could eventually lead to equal deposition of excitation energy within the structure, thus negating the nonlinear cross-excitation mechanism. However, even in the limit of strong coupling, more complex antenna designs may be constructed with modes that are associated with energy localization at specific positions in the design, and which would allow to spatially decouple excitation and readout in a similar way as shown here. In addition, methods of nonlinear cross-excitation may be combined with shaping the incident light field itself [39] , [40] to achieve nanoscale focusing of energy inside the plasmonic nanostructure and enable a new class of reconfigurable optical nanocircuits. In conclusion, we have demonstrated resonant excitation of an ultrafast nonlinearity through a plasmonic hotspot. Using arrays of dimer antennas, we have shown that resonant pumping provides up to four times increase of the nonlinear response of both fast, nonthermal contributions from the external Kerr medium and slow, thermal effects intrinsic to the metal antennas. The two contributions could be independently controlled by using arrays of crossed antennas, where it was shown that the fast, nonthermal effect was efficiently transferred from the pumped antenna to the readout antenna through a hotspot-mediated nonlinearity of the substrate. In comparison, the slow, thermal response, contained mainly in the pumped antenna, was not transferred across the gap, resulting in a reduction of hot electron and thermal contributions in the readout signal. The separation of different types of nonlinear response based on their characteristic dependence on wavelength, time dynamics and antenna geometry is of interest for a next generation of devices aimed at active control of the flow and emission of light in nanoscale optical circuits. Fabrication of nanoantennas Arrays of gold nanoantennas consisting of four arms at right angles were fabricated using e-beam lithography (JEOL JBX-9300FS) at 100 keV with a dose of 650 μC cm −2 on an ITO-coated commercially available substrate (Sigma-Aldrich, sheet resisitivity of 8–12 Ω −2 ), with varying arm lengths in vertical direction. After development, 20 nm of gold was evaporated followed by lift off in acetone. The width of the antenna arms was fixed at 80 nm. Optical experiments Spectral characterization of the nanoantenna transmission was performed using an ytterbium fibre laser amplifier (Fianium, Ltd.) over a spectral range of 500–1,800 nm. Wavelength selection was implemented by a subtractive double prism monochromator. Femtosecond nonlinear pump–probe spectroscopy was done using a regenerative amplified laser system (Pharos/Orpheus) at 10 kHz modulation freqency. The idler of the Orpheus OPA was used as the probe signal in the wavelength range 1,100–1,800 nm and the output from the amplifier at either 1,030 nm or at its second harmonic at 515 nm was used as pump excitation. The pump energy used amounted to 40 nJ per pulse, which was focused to a spot of ~30 μm radius, yielding a fluence on the sample of 4 mJ cm −2 . A signal-to-noise ratio of around 10 −4 Hz −1/2 was obtained by lock-in detection of a modulation of the pump achieved using a mechanical chopper. A small thermal background was subtracted from the spectral maps of Figs 1d,e and 3b–d to highlight the ultrafast response. A large background intensity was only observed for horizontal pump polarization and was indicative of a significant direct heating of the readout antenna by the pump absorption. Simulations Full electrodynamical calculations of the optical response were performed using the finite element method (Comsol 4.3b), taking into account the substrate and the fine details of the antenna geometry. The nanorods were filleted off on a radius of 50 nm. The width of the unit cell as well as the horizontally aligned nanorod were kept the same, while the vertical nanorod and the height of the unit cell were increased in accordance with the experimental parameters. The hotspots where the nonlinear cross-coupling was mediated were modelled by intersecting the ITO layer with a sphere of 150 nm diameter. The absorption cross-sections of the nanoantennas were obtained by calculating the volume integral over the total power dissipation density inside the objects. How to cite this article: Abb, M. et al . Hotspot-mediated ultrafast nonlinear control of multifrequency plasmonic nanoantennas. Nat. Commun. 5:4869 doi: 10.1038/ncomms5869 (2014).